Splicing factor SRSF3 is crucial for hepatocyte differentiation and metabolic function SR family RNA binding proteins regulate splicing of nascent RNAs in vitro but their physiological role in vivo is largely unexplored, as genetic deletion of many SR protein genes results in embryonic lethality. Here we show that SRSF3HKO mice carrying a hepatocyte-specific deletion of Srsf3 (homologous to human SRSF3/SRp20) have a disrupted hepatic architecture and show pre- and postnatal growth retardation. SRSF3HKO mice exhibit impaired hepatocyte maturation with alterations in glucose and lipid homeostasis characterized by reduced glycogen storage, fasting hypoglycemia, increased insulin sensitivity and reduced cholesterol synthesis. We identify various splicing alterations in the SRSF3HKO liver that explain the in vivo phenotype. In particular, loss of SRSF3 causes aberrant splicing of Hnf1 α, Ern1 , Hmgcs1 , Dhcr7 and Scap genes, which are critical regulators of glucose and lipid metabolism. Our study provides the first evidence for a SRSF3-driven genetic programme required for morphological and functional differentiation of hepatocytes that may have relevance for human liver disease and metabolic dysregulation. SRSF3 (previously known as SRp20) is the smallest member of the arginine-serine-rich (SR) proteins family of RNA binding proteins that were originally identified through their ability to alter splicing of pre-mRNAs [1] , [2] , [3] . More recently, SR proteins have been shown to have multiple additional roles in RNA metabolism including transcription, termination, polyadenylation, export, translation and degradation [4] , [5] , [6] , [7] . Although SR proteins are collectively essential for splicing, individual SR proteins do exhibit unique substrate specificities and recognize distinct cis -acting splicing elements in pre-mRNA [8] , [9] . Individual SR proteins also have different tissue distributions [10] , [11] , suggesting potential cell-specific roles in the development and specification of cell lineages. Given the essential roles that SR proteins play in coupling transcriptional and post-transcriptional events in gene expression, one might expect that defects in these processes would lead to developmental impairments and disease pathophysiology. Indeed, dysregulated expression of splicing factors is seen in a number of diseases, such as myotonic dystrophy [12] , [13] and cancer [14] , [15] , underscoring the importance of correct RNA splicing for normal cellular function [16] , [17] . Although SR proteins and related splicing regulators have been studied extensively at the biochemical and cell biological level, relatively little is known about their functions in vivo [18] , [19] and how they contribute to metabolism and development. The analysis of complete genetic deletions is complicated by the observation that null mutations in many SR proteins cause embryonic lethality [20] , [21] , [22] . Indeed, genetic deletion of SRSF3 prevents blastocyst formation, causing death of preimplantation embryos at the morula stage [23] . The blastocyst is the first developmental stage with known differentiated cell lineages, suggesting that SRSF3 is essential for initiating this early genetic programme. SRSF3 is also essential for later developmental decisions such as those in B-cell development [24] . Our previous work demonstrated that SRSF3 regulates splicing of the insulin receptor ( INSR ) gene in hepatoma cells [25] promoting inclusion of exon 11 that encodes 12 amino acids in the ligand-binding domain. As the liver INSR is essential for the correct regulation of glucose and lipid metabolism [26] , we generated a mouse model with a hepatocyte-specific deletion of the Srsf3 gene (SRSF3HKO mice) to define the role of SRSF3 in hepatic function in vivo. Here we report a striking phenotype associated with SRSF3 ablation in hepatocytes. Detailed molecular analysis showed that SRSF3 is a master regulator of hepatic gene expression in the early postnatal period and is essential for hepatic maturation and metabolic function as the SRSF3HKO mice show disturbed hepatic architecture and alterations in glucose and lipid metabolism. SRSF3HKO mice show altered hepatic architecture The SRSF3HKO mice were generated by breeding Srsf3 -floxed and albumin-cre mice as described in Methods. Srsf3 deletion is specific to the liver and is not seen in other tissues ( Supplementary Fig. S1 ). Quantitative PCR (qPCR) results showed that hepatic Srsf3 mRNA is decreased by 70% and primary hepatoctyes do not express SRSF3 protein ( Supplementary Fig. S1c ,d). SRSF3HKO livers show partial skipping of Insr exon 11, confirming our in vitro observations on the human INSR gene [25] ( Supplementary Fig. S1e ). SRSF3HKO pups are obtained at a lower than the expected Mendelian ratio with only 17 knockout mice being obtained at weaning out of 277 total pups, compared with 165 for cre-negative control litters ( Supplementary Table S1 ), and examination revealed that pups are significantly smaller than wild-type (WT) littermates at 2 days of age and many die perinatally. Whole body histological sections show impaired thymic and kidney development, and reduced brown adipose tissue ( Supplementary Fig. S2a ,b). The surviving SRSF3HKO mice have significantly reduced body and liver mass at 1 month of age ( Fig. 1a–c ). Morphologically the SRSF3HKO livers are smaller and paler than WT livers with a roughened surface and multiple small nodules ( Fig. 1d ). The liver mass to body mass ratio is also reduced ( Fig. 1e ). Examination of liver sections revealed a disturbed architecture with large irregular hepatocytes, compressed sinusoidal spaces and bile canaliculi, and clusters of small haematopoietic cells ( Fig. 1f ). At higher magnification control livers show regularly sized hepatocytes with small round nuclei and many bi-nucleated cells ( Fig. 1g ), but hepatocytes in SRSF3HKO livers are larger with irregularly sized nuclei and dense mitotic figures. These observations suggest alterations in cell cycle control and, indeed, SRSF3HKO livers stain positive for both proliferative markers such as Ki67 ( Fig. 1h ) and PCNA ( Supplementary Fig. S3a ) and also for apoptosis by TdT-mediated dUTP nick end labelling (TUNEL) ( Fig. 1i ). Quantification showed a 30% increase in apoptosis in the SRSF3 HKO livers ( Supplementary Fig. S3b ). Consistent with increased cell death, SRSF3 HKO mice show very high serum alanine aminotransferase, alkaline phosphatase and aspartate aminotransferase levels ( Fig. 1j ). Total serum protein is decreased due to a 30% decrease in serum albumin, and bilirubin is increased, but blood urea nitrogen, calcium and creatinine are normal indicating normal kidney function ( Supplementary Table S2 ). 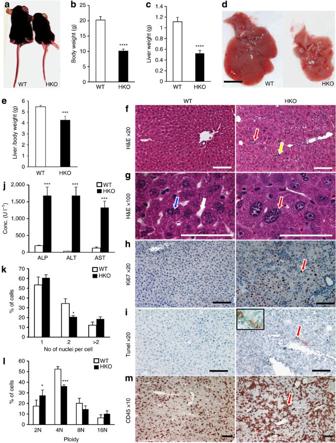Figure 1: SRSF3HKO mice show overall growth retardation and altered hepatic architecture. (a) Representative photograph showing WT mice and SRSF3HKO littermates. (b,c) Body and liver weights for 1-month-old mice;n=7–11. (d) Macroscopic appearance of livers from WT and SRSF3HKO mice. Scale bar, 0.5 cm. (e) Liver to body weight ratio for WT and SRSF3HKO mice;n=7–11. (f,g) Microscopic liver morphology by haematoxylin and eosin (H&E) staining. Yellow arrow shows a cluster of haematopoetic cells present in SRSF3HKO liver. At higher magnification (X100), blue arrow indicates a binuclear cell and white arrow indicates a sinusoid. Red arrow indicates cells with large irregular nuclei. (h) Ki67 staining; red arrow indicates Ki67-positive nuclei in SRSF3HKO liver. (i) TUNEL staining; red arrow shows TUNEL-positive cells in SRSF3HKO liver; inset shows enlargement of apoptotic cells. (j) Serum liver enzymes in WT and SRSF3HKO mice. (k) Quantification of number of nuclei per hepatocyte by laser-scan cytometry. (l) Quantitative analysis of hepatocyte DNA content (ploidy) by flow cytometry;n=3. (m) CD45 immunostaining for haematopoietic cells; red arrow indicates CD45-positive cells. In all images scale bar, 100 μm. Results are means±s.e.m. For panels (j,k),n=4; *P<0.05, ***P<0.001 and ****P<0.0001. Figure 1: SRSF3HKO mice show overall growth retardation and altered hepatic architecture. ( a ) Representative photograph showing WT mice and SRSF3HKO littermates. ( b , c ) Body and liver weights for 1-month-old mice; n =7–11. ( d ) Macroscopic appearance of livers from WT and SRSF3HKO mice. Scale bar, 0.5 cm. ( e ) Liver to body weight ratio for WT and SRSF3HKO mice; n =7–11. ( f , g ) Microscopic liver morphology by haematoxylin and eosin (H&E) staining. Yellow arrow shows a cluster of haematopoetic cells present in SRSF3HKO liver. At higher magnification (X100), blue arrow indicates a binuclear cell and white arrow indicates a sinusoid. Red arrow indicates cells with large irregular nuclei. ( h ) Ki67 staining; red arrow indicates Ki67-positive nuclei in SRSF3HKO liver. ( i ) TUNEL staining; red arrow shows TUNEL-positive cells in SRSF3HKO liver; inset shows enlargement of apoptotic cells. ( j ) Serum liver enzymes in WT and SRSF3HKO mice. ( k ) Quantification of number of nuclei per hepatocyte by laser-scan cytometry. ( l ) Quantitative analysis of hepatocyte DNA content (ploidy) by flow cytometry; n =3. ( m ) CD45 immunostaining for haematopoietic cells; red arrow indicates CD45-positive cells. In all images scale bar, 100 μm. Results are means±s.e.m. For panels ( j , k ), n =4; * P <0.05, *** P <0.001 and **** P <0.0001. Full size image Binuclearity is a marker of hepatocyte maturation [27] , [28] . Inspection of haematoxylin and eosin-stained tissue sections suggested that fewer cells were binuclear in the SRSF3HKO livers ( Fig. 1g ). Analysis of primary hepatocytes by laser-scan cytometry confirmed that the percentage of bi-nuclear cells is indeed reduced in SRSF3HKO livers ( Fig. 1k ) and also confirmed the heterogeneity in hepatocyte size ( Supplementary Fig. S4a ). This finding was independently verified by flow cytometry ( Fig. 1l and Supplementary Fig. S4b ) that showed decreased tetraploid and increased diploid cells in SRSF3HKO livers consistent with the reduced bi-nuclearity. The increased expression of proliferative markers, reduced number of binuclear hepatocytes and tetraploidy, and the presence of haematopoetic cells suggested impaired hepatic differentiation and maturation. Sections of livers from 2-day-old pups show haematopoietic cells in both WT and SRSF3HKO livers ( Supplementary Fig. S2c ) consistent with haematopoiesis in the fetal liver [29] . Although WT livers show only residual CD45-positive haematopoietic cells at 1 month, the SRSF3HKO livers show continued presence of haematopoietic cells ( Fig. 1m ). The normal numbers of circulating blood cells ( Supplementary Table S3 ) confirms a defect in hepatocyte maturation rather than a compensatory increase in extramedullary haematopoiesis due to anaemia. Furthermore, the altered hepatocyte proliferation and apoptosis might be expected to impair liver repair; however, the regenerative capacity of the liver is unaffected as both genotypes show a similar proliferative response after partial hepatectomy ( Supplementary Fig. S5 ). Loss of SRSF3 causes impaired glucose homeostasis The previous data pointed to a defect in hepatocyte maturation that was confirmed by analysing selected gene expression. Livers from SRSF3HKO mice showed dramatic upregulation of the fetal markers alpha-fetoprotein and H19 mRNA expression and downregulation of the mature marker albumin ( Alb ) compared with WT mice at 1 month of age ( Fig. 2a ). Silencing of Srsf3 in adult liver by AAV-mediated cre-recombination caused a similar phenotype of increased H19 expression and increased apoptosis indicating that the phenotype is likely due to de-differentiation ( Supplementary Fig. S6 ). 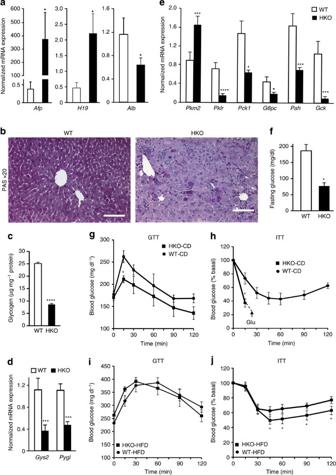Figure 2: Effect of hepatic SRSF3 KO on gene expression and metabolic markers. (a) mRNA expression of fetal markers alpha-fetoprotein (Afp)andH19and adult liver markerAlb;n=5–8. (b) Periodic acid-Schiff (PAS) staining for liver glycogen (magenta colour). Scale bar, 100 μm. (c) Biochemical measurement of glycogen levels in WT and SRSF3HKO liver;n=8. (d) mRNA expression of glycogen synthase (Gys2) and glycogen phosphorylase (Pygl) in SRSF3HKO and WT mice;n=4–6. (e) Metabolic enzyme mRNA expression forPkm2,Pklr,Pck1,G6pc,PahandGckby qPCR;n=4–8. (f) Fasting blood glucose levels in 1–month-old SRSF3HKO and WT mice.n=3–4 (g) Blood glucose concentrations during GTT on 4-month-old mice fed a low-fat, control diet for 12 weeks. (h) Blood glucose concentrations during an ITT for 4-month-old mice fed a low-fat, control diet for 12 weeks. Arrow indicates when mice were rescued by an i.p. bolus injection of glucose to reverse severe hypoglycemic shock.n=3–6 forgandh. (i) Blood glucose concentrations during GTT for 4-month-old mice fed HFD for 12 weeks. (j) Blood glucose concentrations during an ITT for 4-month-old mice fed HFD for 12 weeks.n=4–8 foriandj. Results are means±s.e.m. *P<0.05, ***P<0.001, ****P<0.0001. Figure 2: Effect of hepatic SRSF3 KO on gene expression and metabolic markers. ( a ) mRNA expression of fetal markers alpha-fetoprotein ( Afp) and H19 and adult liver marker Alb ; n =5–8. ( b ) Periodic acid-Schiff (PAS) staining for liver glycogen (magenta colour). Scale bar, 100 μm. ( c ) Biochemical measurement of glycogen levels in WT and SRSF3HKO liver; n =8. ( d ) mRNA expression of glycogen synthase ( Gys2 ) and glycogen phosphorylase ( Pygl ) in SRSF3HKO and WT mice; n =4–6. ( e ) Metabolic enzyme mRNA expression for Pkm2 , Pklr , Pck1 , G6pc , Pah and Gck by qPCR; n =4–8. ( f ) Fasting blood glucose levels in 1–month-old SRSF3HKO and WT mice. n =3–4 ( g ) Blood glucose concentrations during GTT on 4-month-old mice fed a low-fat, control diet for 12 weeks. ( h ) Blood glucose concentrations during an ITT for 4-month-old mice fed a low-fat, control diet for 12 weeks. Arrow indicates when mice were rescued by an i.p. bolus injection of glucose to reverse severe hypoglycemic shock. n =3–6 for g and h . ( i ) Blood glucose concentrations during GTT for 4-month-old mice fed HFD for 12 weeks. ( j ) Blood glucose concentrations during an ITT for 4-month-old mice fed HFD for 12 weeks. n =4–8 for i and j . Results are means±s.e.m. * P <0.05, *** P <0.001, **** P <0.0001. Full size image Glycogen staining by periodic acid-Schiff reagent is noticeably weaker in sections of HKO livers and biochemical quantification showed a 60% decrease in stored glycogen ( Fig. 2b ). The decrease in hepatic glycogen was associated with decreases in expression of both Gys2 and Pygl , the major isoforms of glycogen synthase and glycogen phosphorylase in the liver ( Fig. 2d ). Furthermore, the SRSF3HKO liver showed elevated expression of the fetal isozyme of pyruvate kinase 2 ( Pkm2 ) and, conversely, decreased expression of several metabolic enzymes that are characteristic of mature hepatocytes including the L-isozyme of pyruvate kinase ( Pklr ), glucokinase ( Gck ), phosphoenolpyruvate carboxykinase ( Pck1 ), glucose-6-phosphatase ( G6pc ) and phenyl-alanine hydroxylase ( Pah ) ( Fig. 2e ). The alterations in glycogen and gluconeogenic enzymes suggested that the mice might have defective hepatic glucose production and, indeed, SRSF3HKO mice showed fasting-induced hypoglycemia at 1 month of age, although there was no difference in fasting insulin levels compared with WT animals ( Fig. 2f and Supplementary Table S2 ). By 4 months of age the SRSF3HKO mice weighed the same as WT littermates ( Supplementary Fig. S7 ) and fasting blood glucose levels were normal. Glucose tolerance tests performed on 4-month-old SRSF3HKO mice that had been maintained on a standard low-fat chow diet for 12 weeks showed decreased glucose at 15 min but the values at subsequent times were indistinguishable from WT mice. This suggests that suppression of hepatic glucose production is more pronounced in SRSF3HKO mice but that peripheral glucose uptake into muscle and fat at later times is not altered ( Fig. 2g ). Subsequent insulin tolerance tests (ITT) demonstrated increased insulin sensitivity and an inability to correct insulin-induced hypoglycemia. Insulin treatment caused a very rapid drop in blood glucose levels in SRSF3HKO mice at 15 min and the mice showed signs of severe hypoglycemia and had to be rescued with glucose injections ( Fig. 2h ). In parallel, a second cohort of mice were maintained on a 60% high-fat diet (HFD) for 12 weeks to determine the effect of lipid overload on glucose metabolism. Although the SRSF3HKO mice were initially lighter than WT littermates, they showed compensatory weight gain on both control and HFD ( Supplementary Fig. S7 ). As expected, the HFD caused glucose intolerance and insulin resistance in the WT mice and also in the SRSF3HKO mice ( Fig. 2i ). SRSF3HKO mice again showed increased insulin sensitivity compared with the WT littermates with a greater drop in blood glucose during the ITT expansion for ITT provided before. ( Fig. 2j ). Taken together, these results indicated that hepatocyte maturation is compromised and hepatic glucose production is impaired in SRSF3HKO liver resulting in relative insulin sensitivity. Altered splicing and gene expression in SRSF3HKO liver To understand how loss of SRSF3 alters hepatocyte maturation and metabolism, we performed microarray analyses of gene expression and exon utilization. Deletion of Srsf3 caused a dramatic alteration in gene expression in the liver ( Fig. 3a ). To identify the most robust changes in gene expression and exon utilization, array data was analysed by multiple statistical approaches as described in Supplementary Methods . Analysis of the array data for changes in exon utilization indicated that 956 genes showed evidence for significantly altered exon use ( Supplementary Data 1 ) and Gene Ontology analysis indicated that these genes are involved in development, immune response, lipid metabolism and cytoskeleton and cell adhesion ( Fig. 3b ). Analysis of enriched pathways and processes indicated that the aberrantly spliced genes are involved in fatty acid metabolism and oxidation, the immune response, development, angiogenesis and the unfolded protein/ER endoplasmic reticulum stress response (UPR) ( Supplementary Tables S4 and S5 ). 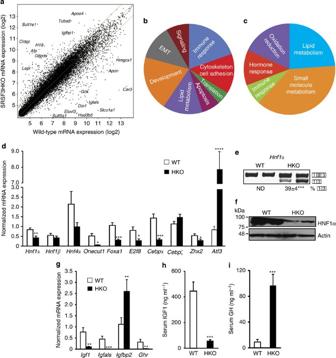Figure 3: Altered gene expression and GH resistance in SRSF3HKO mice. (a) Scatterplot of normalized mRNA expression by microarray. Data are log2 normalized. Some of the most highly up- or downregulated genes are indicated. (b) Gene ontology mapping of genes that show significantly altered splicing. (c) Gene ontology mapping of genes that show significantly altered expression. (d) mRNA expression of selected liver transcription factors by qPCR;n=8. (e) Analysis ofHnf1α exon 2 splicing by RT–PCR. A representative gel is shown with two WT and SRSF3HKO samples with the percentage of exon skipping indicated underneath. ND, not detectable. (f) HNF1α protein expression in hepatocyte lysates by immunoblotting with two representative animals per group. Blots were stripped and reblotted for actin as a loading control. (g) mRNA expression of the known HNF1α target genesIgf1,Igfals,Igfbp2andGhr, in SRSF3HKO and WT liver by qPCR.n=8 (h) Total serum IGF1 in SRSF3HKO and WT mice.n=7 (i) Serum GH in SRSF3HKO and WT mice.n=8. Results are means±s.e.m. In all panels,nindicates the number of mice per group, *P<0.05, **P<0.01, ***P<0.001, ****P<0.0001. Figure 3: Altered gene expression and GH resistance in SRSF3HKO mice. ( a ) Scatterplot of normalized mRNA expression by microarray. Data are log2 normalized. Some of the most highly up- or downregulated genes are indicated. ( b ) Gene ontology mapping of genes that show significantly altered splicing. ( c ) Gene ontology mapping of genes that show significantly altered expression. ( d ) mRNA expression of selected liver transcription factors by qPCR; n =8. ( e ) Analysis of Hnf1 α exon 2 splicing by RT–PCR. A representative gel is shown with two WT and SRSF3HKO samples with the percentage of exon skipping indicated underneath. ND, not detectable. ( f ) HNF1α protein expression in hepatocyte lysates by immunoblotting with two representative animals per group. Blots were stripped and reblotted for actin as a loading control. ( g ) mRNA expression of the known HNF1α target genes Igf1 , Igfals , Igfbp2 and Ghr , in SRSF3HKO and WT liver by qPCR. n =8 ( h ) Total serum IGF1 in SRSF3HKO and WT mice. n =7 ( i ) Serum GH in SRSF3HKO and WT mice. n =8. Results are means±s.e.m. In all panels, n indicates the number of mice per group, * P <0.05, ** P <0.01, *** P <0.001, **** P <0.0001. Full size image The microarrays also identified significant expression changes for 895 genes ( Supplementary Data 2 ) and Gene Ontology analysis revealed that these genes are involved in lipid and small molecule metabolism ( Fig. 3c ). The enriched biological pathways were cholesterol and steroid biosynthesis and the enriched disease and toxicity pathways were dyslipidemia, insulin resistance, cholestasis and steatosis ( Supplementary Tables S6 and S7 ). We subjected the list of altered genes to a de novo network analysis to uncover the transcription factors driving gene expression, which revealed that the liver-enriched factors HNF1α, HNF4α, C/EBPβ and SREBP1 are among the top transcription factors regulating these genes ( Supplementary Table S8 ). An interactome analysis showed that HNF1α, SREBP1, HNF4α, SREBP2, HNF3β (FoxA2), C/EBPβ and HNF1β are among the top over-connected transcription factors similar to the network analysis ( Supplementary Table S8 ). Loss of SRSF3 causes growth hormone resistance Given the importance of liver-enriched transcription factors in our network analysis, changes in expression of selected transcription factors were assessed by qPCR. The expression of Hnf1 α, Hnf6 α ( Onecut1 ), Foxa1 ( Hnf3 α), E2F8 , Zhx2 , C/EBP α, was significantly decreased in SRSF3HKO liver but Hnf1 β, Hnf4 α and C/EBP ζ were not changed and Atf3 was increased ( Fig. 3d ). Exon utilization data also indicated a novel aberrant splicing event in the Hnf1 α gene in SRSF3HKO liver. Reverse transcription PCR (RT–PCR) analysis confirmed that the exon 2 of Hnf1 α was partially skipped ( Fig. 3e ) in SRSF3 HKO liver. Skipping of exon 2 will introduce a premature termination codon (PTC) in the Hnf1 α transcript, which should trigger non-sense-mediated decay. This explains the observed reduction in both Hnf1 α transcripts and HNF1α protein in SRSF3HKO liver ( Fig. 3f ). Hence, SRSF3 is required for proper exon utilization and expression of HNF1α in postnatal mouse liver. As a result of decreased HNF1α expression, the target genes Ghr , Igf1 and Igfals were also reduced ( Fig. 3g ), and consequently SRSF3HKO mice show decreased serum insulin-like growth factor 1 (IGF1) but increased serum growth hormone (GH) indicating GH insensitivity ( Fig. 3h ). Hepatic cholesterol is reduced in SRSF3HKO liver The transcriptome data indicated that multiple genes in cholesterol biosynthesis are reduced ( Supplementary Fig. S8 ). A number of cholesterol biosynthetic genes are direct targets for SRSF3, as splicing of 3-hydroxy-3-methylglutaryl-CoA synthase 1 ( Hmgcs1 ) and 7-dehydrocholesterol reductase ( Dhcr7 ) are altered in SRSF3HKO liver ( Fig. 4a ). Also, the SREBP cleavage activating protein ( Scap ) gene, which activates SREBP2, shows aberrant splicing with partial skipping of exon 17 and retention of introns 13 and 14 ( Fig. 4b ). All three aberrantly-spliced genes are also significantly downregulated as are Srebp1 and Srebp2 ( Fig. 4c ). As a result, processing of SREBP2 is reduced ( Fig. 4d ) and the SREBP2 target genes, Hmgcr , Mvk , Pmvk , Mvd , Fdpt1 and Sqle/Erg1 in the cholesterol biosynthetic pathway are decreased in SRSF3HKO liver. 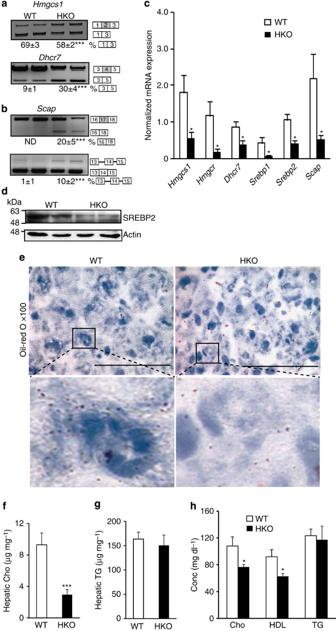Figure 4: Hepatic and serum cholesterol is reduced in SRSF3HKO liver at 1 month of age. (a) Analysis of exon skipping inHmgcs1andDhcr7transcripts. A representative gel is shown with two WT and SRSF3HKO samples with the percentage of exon skipping underneath. (b) Analysis of exon skipping (upper panel) and intron retention (lower panel) inScaptranscripts. A representative gel is shown with two WT and SRSF3HKO samples with the percentage of exon skipping/intron retention. ND, not detectable. (c) mRNA expression ofHmgcs1,Hmgcr,Dhcr7,Srebp1,Srebp2andScapin WT and SRSF3HKO liver by qPCR;n=8. (d) SREBP2 protein expression in hepatocyte lysates by immunoblotting with two representative animals per group. Blots were stripped and reblotted for actin as a loading control. (e) Oil-Red-O staining for lipid droplets in SRSF3HKO and WT livers (upper panel × 100). Lower panel shows enlargement of boxed region in upper panel. Scale bar, 100 μm. (f) Hepatic cholesterol in SRSF3HKO and WT mice.n=8–10 (g) Hepatic TGs in SRSF3HKO and WT mice.n=7–12 (h) Circulating cholesterol (Cho), high-density lipoprotein (HDL) and TGs in SRSF3HKO and WT mice;n=3–4. Results are means±s.e.m. In all panels,nindicates the number of mice per group, *P<0.05 and ***P<0.001. Figure 4: Hepatic and serum cholesterol is reduced in SRSF3HKO liver at 1 month of age. ( a ) Analysis of exon skipping in Hmgcs1 and Dhcr7 transcripts. A representative gel is shown with two WT and SRSF3HKO samples with the percentage of exon skipping underneath. ( b ) Analysis of exon skipping (upper panel) and intron retention (lower panel) in Scap transcripts. A representative gel is shown with two WT and SRSF3HKO samples with the percentage of exon skipping/intron retention. ND, not detectable. ( c ) mRNA expression of Hmgcs1 , Hmgcr , Dhcr7 , Srebp1 , Srebp2 and Scap in WT and SRSF3HKO liver by qPCR; n =8. ( d ) SREBP2 protein expression in hepatocyte lysates by immunoblotting with two representative animals per group. Blots were stripped and reblotted for actin as a loading control. ( e ) Oil-Red-O staining for lipid droplets in SRSF3HKO and WT livers (upper panel × 100). Lower panel shows enlargement of boxed region in upper panel. Scale bar, 100 μm. ( f ) Hepatic cholesterol in SRSF3HKO and WT mice. n =8–10 ( g ) Hepatic TGs in SRSF3HKO and WT mice. n =7–12 ( h ) Circulating cholesterol (Cho), high-density lipoprotein (HDL) and TGs in SRSF3HKO and WT mice; n =3–4. Results are means±s.e.m. In all panels, n indicates the number of mice per group, * P <0.05 and *** P <0.001. Full size image Consistent with impaired lipid synthesis, Oil-Red-O staining showed fewer lipid droplets in sections of 1-month-old SRSF3HKO liver ( Fig. 4e ) and biochemical analysis showed that this is due to reduced cholesterol rather than triglyceride (TG) ( Fig. 4f ). Serum cholesterol and high-density lipoprotein are also lower ( Fig. 4h ), consistent with the hepatic levels at this age. Alterations in lipid metabolism were also seen in 4-month-old mice that had been maintained on control or HFD for 15 weeks. Sections of livers of both SRSF3HKO and WT mice on HFD showed hepatic steatosis ( Fig. 5a ) and total body fat was increased, although the SRSF3HKO mice were slightly leaner ( Fig. 5b ). WT mice showed increased hepatic TG but, surprisingly, the SRSF3HKO mice on the control diet also showed increased hepatic TG that did not increase on HFD ( Fig. 5c ). Serum TG is lower in SRSF3HKO mice on control diet but is unchanged on HFD ( Fig. 5d ). Unlike the younger mice, hepatic cholesterol was not altered at 4 months of age ( Fig. 5e ) and serum cholesterol was increased by HFD in both SRSF3HKO and WT mice although the levels were consistently lower in the SRSF3HKO mice ( Fig. 5f ). 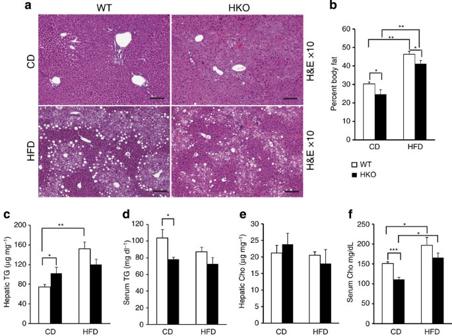Figure 5: TGs and cholesterol are altered in SRSF3HKO mice at 4 months of age. (a) Haematoxylin and eosin (H&E)-stained liver sections for WT and SRSF3HKO mice fed low-fat, control diet (CD, upper panel) or HFD (lower panel) for 12 weeks starting at 4 weeks of age. Scale bar, 100 μm. (b) Total body fat measured by DEXA scanning in SRSF3HKO or WT mice fed control diet and HFD for 12 weeks. (c,d) Hepatic and serum TGs in SRSF3HKO (black) and WT mice (white) after 12 weeks. (e,f) Hepatic and serum cholesterol in HKO and WT mice after 12 weeks. Results are means±s.e.m. In all panels,n=2–8 mice per group, *P<0.05, **P<0.01, ***P<0.001. Figure 5: TGs and cholesterol are altered in SRSF3HKO mice at 4 months of age. ( a ) Haematoxylin and eosin (H&E)-stained liver sections for WT and SRSF3HKO mice fed low-fat, control diet (CD, upper panel) or HFD (lower panel) for 12 weeks starting at 4 weeks of age. Scale bar, 100 μm. ( b ) Total body fat measured by DEXA scanning in SRSF3HKO or WT mice fed control diet and HFD for 12 weeks. ( c , d ) Hepatic and serum TGs in SRSF3HKO (black) and WT mice (white) after 12 weeks. ( e , f ) Hepatic and serum cholesterol in HKO and WT mice after 12 weeks. Results are means±s.e.m. In all panels, n =2–8 mice per group, * P <0.05, ** P <0.01, *** P <0.001. Full size image Loss of SRSF3 dysregulates the unfolded protein response Aberrant splicing results in PTCs due to exon skipping or intron retention, and translation of these aberrant mRNAs often leads to misfolded proteins that induce the UPR. Inspection of UPR-related genes revealed altered splicing of both the Ern1 gene, which encodes the inositol-requiring enzyme 1α (IRE1α) and its downstream target gene Xbp1 that encodes the transcription factor X-box binding protein 1 (XBP1) ( Fig. 6a and Supplementary Data 1 ). Exon 13 was skipped in 71% of Ern1 transcripts in SRSF3HKO liver ( Fig. 6a ) and transcripts lacking exon 13 are predicted to produce a PTC before the ribonuclease domain encoded in exon 14 and produce a nonfunctional protein. Consequently, splicing of Xbp1 was also impaired and the expression of both IRE1α and spliced XBP1 proteins was reduced ( Fig. 6b ). Consistent with reduced XBP1 expression, the UPR genes ER degradation-enhancing alpha-mannosidase-like 1 ( Edem1 ) and catalase ( Cat ) were significantly downregulated in SRSF3HKO liver as were the XBP1-dependent lipogenic genes Scd1 , Dgat2 and Acc2 ( Fig. 6c ). The reduction in lipogenic genes but normal or elevated hepatic TG levels suggested that fatty acid metabolism might be reduced. Indeed, measurement of fatty acid oxidation on liver extracts from SRSF3HKO mice revealed a significant decrease compared with WT mice ( Fig. 6d ). 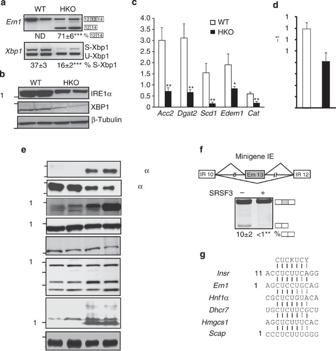Figure 6: Loss of SRSF3 dysregulates the UPR. (a) Analysis ofXbp1andErn1splicing. A representative gel is shown with two WT and two SRSF3HKO samples and the percentage of exon 13 skipping forErn1and splicedXbp1(S-Xbp1) is shown below.S-Xbp1andU-Xbp1indicate the spliced and unspliced form ofXbp1, respectively. (b) XBP1 and IRE1α protein expression by immunoblotting. Blots were stripped and reblotted for β-tubulin. (c) mRNA expression of XBP1 target genesAcc2,Dgat2,Scd1,Edem1andCatin SRSF3HKO and WT mice by qPCR;n=8. (d) Fatty acid oxidation in liver lysates from SRSF3HKO and WT mice;n=3–4. (e) eIF2α and PERK phosphorylation, GRP78 and GRP94 expression, and ATF6 and caspase-3 processing and cleavage measured by immunoblotting SRSF3HKO and WT liver lysates. Blots were stripped and reblotted for eIF2α and actin as loading controls. (f) Schematic drawing of a minigene containingINSRexons 10 and 12 (white boxes) andErn1exon 13 (grey box). Representative gel shows exon 13 skipping in RNA from NIH3T3 cells transfected with the minigene with or without a SRSF3 expression plasmid (n=3 expts). (g) Consensus binding motif of SRSF3 is present in exons ofInsr,Ern1,Hnf1α,Dhcr7andScapand also in the downstream exon 3 ofHmgcs1. Results are means±s.e.m. *P<0.05 and **P<0.01, and ***P<0.001. Figure 6: Loss of SRSF3 dysregulates the UPR. ( a ) Analysis of Xbp1 and Ern1 splicing. A representative gel is shown with two WT and two SRSF3HKO samples and the percentage of exon 13 skipping for Ern1 and spliced Xbp1 (S- Xbp1 ) is shown below. S-Xbp1 and U-Xbp1 indicate the spliced and unspliced form of Xbp1 , respectively. ( b ) XBP1 and IRE1α protein expression by immunoblotting. Blots were stripped and reblotted for β-tubulin. ( c ) mRNA expression of XBP1 target genes Acc2 , Dgat2 , Scd1 , Edem1 and Cat in SRSF3HKO and WT mice by qPCR; n =8. ( d ) Fatty acid oxidation in liver lysates from SRSF3HKO and WT mice; n =3–4. ( e ) eIF2α and PERK phosphorylation, GRP78 and GRP94 expression, and ATF6 and caspase-3 processing and cleavage measured by immunoblotting SRSF3HKO and WT liver lysates. Blots were stripped and reblotted for eIF2α and actin as loading controls. ( f ) Schematic drawing of a minigene containing INSR exons 10 and 12 (white boxes) and Ern1 exon 13 (grey box). Representative gel shows exon 13 skipping in RNA from NIH3T3 cells transfected with the minigene with or without a SRSF3 expression plasmid ( n =3 expts). ( g ) Consensus binding motif of SRSF3 is present in exons of Insr , Ern1 , Hnf1 α, Dhcr7 and Scap and also in the downstream exon 3 of Hmgcs1 . Results are means±s.e.m. * P <0.05 and ** P <0.01, and *** P <0.001. Full size image In contrast, processing of ATF6 is increased and PERK and eIF2α are constitutively phosphorylated in both SRSF3HKO liver extracts ( Fig. 6e ) and primary hepatocytes (data not shown), suggesting that the other arms of the UPR are activated. Furthermore, Atf4 [30] , [31] (refs 30 , 31 ) and its target genes Ddit3 ( Chop/Gadd153 ) and Atf3 were also significantly increased in SRSF3HKO liver ( Supplementary Data 2 ) but GRP78 and GRP94 levels were unchanged ( Fig. 6e ). Electron microscopy studies revealed dilated RERs consistent with global ER stress ( Supplementary Fig. S9 ). These data indicate that Srsf3 deletion in the liver leads to selective downregulation of the lipogenic IRE1α-XBP1 pathway but upregulation of the proapoptotic PERK-eIF2α-ATF4 and ATF6 pathways, which may explain the elevated level of cleaved caspase-3 ( Fig. 6e ) and apoptotic staining ( Fig. 1h ) in SRSF3HKO liver. To determine whether SRSF3 regulates splicing of Ern1 exon 13 directly, we constructed a minigene where exon 13 of Ern1 was subcloned into an INSR minigene [32] in place of the SRSF3-dependent exon 11 ( Fig. 6f ). Co-transfection of this minigene with an SRSF3 expression plasmid caused increased incorporation of exon 13 ( Fig. 6f ) indicating that exon 13 contains an SRSF3-dependent splicing enhancer. Indeed, alignment of the alternatively spliced exons from Insr , Ern1 , Hnf1 α, Dhcr7 and Scap identified potential binding sites for SRSF3 consistent with missplicing of these exons in SRSF3HKO liver ( Fig. 6g ). In the current study, we have uncovered a physiological role for SRSF3 in hepatocyte maturation and metabolic function. Although SR proteins have many redundant functions, the SRSF3-dependent functions in liver do not appear to be compensated by other SR family proteins. Loss of SRSF3 leads to prolonged expression of fetal markers, decreased expression of adult markers and the persistence of hepatic haematopoiesis. Liver architecture is disrupted and hepatocytes show reduced binuclearity with irregular nuclei and the expression of both proliferative and apoptotic markers. The SRSF3HKO mice are runted and many die perinatally. Postmortem examination of the anatomy shows immature kidney and thymus development and reduced brown adipose tissue that likely contribute to the perinatal lethality. The surviving mice show fasting hypoglycemia, and are unable to correct insulin-induced hypoglycemia due to reduced glycogen stores and gluconeogenic enzyme gene expression. When stressed with a HFD, the mice become glucose-intolerant and insulin-resistant but are relatively more insulin-sensitive than WT littermates. Hepatocyte maturation and differentiation is maintained by a complex network of transcription factors [33] . The interdependency of these transcription factors, their expression and relative promoter occupancy has been documented during liver development [34] . Many of these liver-enriched factors show changes in expression and splicing in SRSF3HKO liver. Of particular importance for liver maturation the expression of Hnf1α , Onecut1 ( Hnf6 α), Lrh1 , Hhex , Tbx3 , C/ebp α and Foxa2 ( HNF3 β) are all reduced and the fetal transcription factor Gata6 is increased. Some of these genes show changes in splicing as well as expression. In particular, SRSF3HKO livers show aberrant splicing of exon 2 of Hnf1 α creating a PTC before the DNA binding domain. HNF1α has a number of important targets in the liver, including the GH receptor ( Ghr ) gene [35] , and HNF1α-deficient mice have severe growth defects, type 2 diabetes, phenylketonuria, hepatic dysfunction and renal Fanconi syndrome [36] , [37] . SRSF3HKO mice are thus growth hormone-resistant due to loss of HNF1α and decreased expression of Ghr in the liver, with subsequent low circulating IGF-I and elevated GH as is seen in the liver Ghr knockout (GHRLD) mouse [38] . The overall growth defect may not be due to the GH resistance; however, as the GHRLD mouse does not show an overall growth defect. The hepatic knockout of Igf-1 (LID mouse) similarly does not show a growth defect [39] . The GHRLD also shows insulin resistance and glucose intolerance with normal levels of G6pc and Pck1 , serum fatty acids are high due to the lipolytic effect of GH, and the mice show hepatic steatosis [38] . In contrast, the HKO mice are insulin-sensitive and glucose-tolerant with reduced G6pc and Pck1 and normal hepatic and serum TGs and fatty acids but do show reduced adipose tissue, which may reflect elevated GH-mediated lipolysis. The reduced gluconeogenesis could be related to the overexpression of Atf3 in SRSF3HKO mice as Atf3 suppresses Pck1 promoter activity [40] . Genomic analysis identified nearly 1,000 genes with significant evidence for missplicing in SRSF3HKO liver. SRSF3HKO mice show relatively large changes in gene expression and splicing compared with tissue-specific knockouts of other splicing factors such as Rbfox1 in the brain [41] and SRSF1 in the heart [22] , which may lead to a more severe phenotype. An RNA immunoprecipitation (RIP)-chip analysis in p19 neuronal cells identified target genes that are bound by SRSF3 (ref. 42 ). Comparison of these RIP hits reveals that 26% of our misspliced genes are direct targets for SRSF3, the remaining 74% of our misspliced genes may represent genes that are either not expressed in the p19 neuronal cells or are indirect targets. With the aberrant splicing of so many genes, misfolding of mutant proteins might be expected to induce the UPR and, indeed, the PERK-eIF2α and ATF6 pathways are constitutively elevated in SRSF3HKO livers, but the IRE1α-XBP1 pathway was impaired due to the aberrant splicing of Ern1 that effectively blocked the cytoplasmic splicing of Xbp1 . Deletion of Xbp1 or Ern1 is embryonic lethal similar to SRSF3. The Xbp1 embryonic lethality can be rescued by the expression of Xbp1 in the liver whereas IRE1 α is essential for placental development [43] , [44] . Liver-specific deletion of Xbp1 causes a decrease in lipogenic gene expression, decreased hepatic lipid synthesis and secretion, and decreased plasma TGs, cholesterol and free fatty acids without changing the liver architecture [45] . As expected, XBP1-dependent target genes are reduced and the response to ER stress is impaired, but Ddit3 expression is normal, indicating the defect is specific to the XBP1 pathway. Some of the phenotypes in our SRSF3HKO mice can be explained by defects in Xbp1 splicing, in particular the decreased expression of Acc2 , Dgat2 , Scd1 and Fasn are consistent with the Xbp1 liver knockout phenotype and comparison of our data with expression profiling from B cells engineered to overexpress XBP1s highlighted an additional 162 common genes [46] . In contrast, the decreased expression of cholesterol synthetic genes such as Hmgcs1 , Hmgcr , Mvk , Pmvk , Dhcr7 , Erg1 , Fdft1 and Mvd is not seen in the Xbp1 liver knockout. All of these cholesterol biosynthetic genes are regulated by SREBP2, which is activated by SCAP to generate a transcriptionally active N-terminal fragment [47] , [48] . Conditional knockout of Scap in the liver causes an 80% reduction in lipid and cholesterol synthesis [48] . We show here that loss of SRSF3 causes missplicing and decreased expression of Scap , reduced SREBP2 processing and impaired expression of cholesterol biosynthetic genes consistent with the conditional Scap knockout, and comparison of our data with Scap -dependent genes in epithelial cells highlighted a further 37 genes that are co-regulated in both knockouts [49] . Taken together, the results from our SRSF3HKO model indicate that SRSF3 controls the activity of at least three important pathways ( Fig. 7 ). First, the SRSF3-HNF1α-GH-IGF1 pathway that is critical for embryonic and postnatal growth and development. Second, the SRSF3-IRE1α-XBP1 arm of the UPR/ER stress response that regulates hepatic lipogenesis. Third, the SRSF3-SCAP-SREBP2 pathway that controls hepatic cholesterol synthesis. No single mutation or deletion in these pathways is associated with changes in liver architecture and hepatocyte morphology that we observe in our SRSF3HKO mice, so there could be other regulatory pathways that are controlled by SRSF3-dependent splicing events, or the disrupted architecture could result from the cumulative effect of impairment of these individual pathways. In conclusion, our study demonstrates the importance of accurate splicing for liver development, metabolic homeostasis and normal physiology, and lays the groundwork for investigation of dysregulation of splicing factor expression and its contribution to disease pathogenesis. 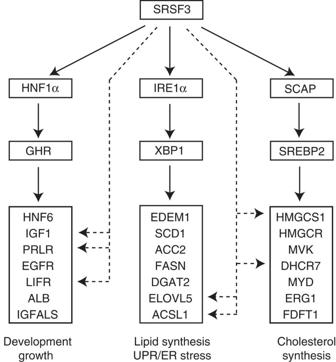Figure 7: SRSF3 controls multiple signalling pathways important for liver homeostasis. Schematic showing downstream genes that are targets for SRSF3 in the mouse hepatocyte. Loss of SRSF3 causes aberrant splicing ofHnf1α,Ern1andScapleading to loss ofGhrexpression,Xbp1splicing and SREBP2 activation, and subsequent loss of downstream target genes that control embryonic growth and liver development, lipid synthesis and ER stress, and cholesterol synthesis, respectively. Dotted lines indicate additional direct targets for SRSF3-dependent splicing. Figure 7: SRSF3 controls multiple signalling pathways important for liver homeostasis. Schematic showing downstream genes that are targets for SRSF3 in the mouse hepatocyte. Loss of SRSF3 causes aberrant splicing of Hnf1 α, Ern1 and Scap leading to loss of Ghr expression, Xbp1 splicing and SREBP2 activation, and subsequent loss of downstream target genes that control embryonic growth and liver development, lipid synthesis and ER stress, and cholesterol synthesis, respectively. Dotted lines indicate additional direct targets for SRSF3-dependent splicing. Full size image Generation of SRSF3HKO mice Srsf3 tm1Pjln mice ( Srsf3flox:flox ) mice are described previously [23] . These mice contain a floxed Srsf3 allele with LoxP sites flanking exons 2 and 3 of Srsf3 , which encode the RNA-binding domain ( Supplementary Fig. S1a ). Floxed Srsf3 mice were mated to TgN ( Alb-Cre ) 21Mgn transgenic mice [50] that express cre recombinase in hepatocytes driven by the rat albumin enhancer/promoter. We crossed the resulting heterozygous Srsf3flox /+; Alb-Cre + mice to Srsf3flox/flox mice to obtain homozygous Srsf3flox/flox;Alb-Cre+ animals (SRSF3HKO) and their control cre-negative littermates. The deleted Srsf3 mRNA was smaller than the WT mRNA due to lack of exon 2 and 3, as confirmed by RT–PCR analysis. One-month-old SRSF3HKO mice and sex-matched SRSF3flox/flox littermates were used as WT controls throughout the study unless otherwise stated. All animal work was reviewed and approved by the University of California San Diego Institutional Animal Care and Use Committee. Diet study Mice were divided into two groups at 5 weeks of age, and were allowed ad libitum access to water and one of the two synthetic diets: a control (low fat) diet and high-fat diet (60% HFD) for 15 weeks. Isolation of primary murine hepatocytes Primary hepatocytes from male WT and SRSF3HKO liver were obtained by two-step perfusion with liver perfusion medium (Gibco BRL 17701-038; Gibco, Detroit, MI) followed by digestion medium, L15 (Sigma L5520; Sigma, St Louis, MO) containing 0.15 g ml −1 collagenase and 10 μg ml −1 DNase I using standard procedure [51] . The liver cells were disaggregated by passing through a 40-μm-pore nylon mesh Cell Strainer (BD Falcon). The numbers of total viable cells were determined by Trypan blue staining. Freshly obtained primary hepatocytes were re-suspended in 1 × PBS to the concentration of 1–2 × 10 6 cells ml −1 and fixed in ethanol. Flow and laser-scanning cytometry Ethanol-fixed hepatocytes were washed with PBS and then stained with 50 μg ml −1 propidium iodide (Sigma) containing 1 mg ml −1 RNase (Sigma) for 30 min at room temperature and analysed by forward-scattering fluorescence-activated cell sorting (FACS) or laser-scanning cytometry to determine cell parameters and DNA content. We repeated these experiments using three biological replicates from SRSF3HKO and WT groups. Cytometry was performed by the Flow Cytometry Research Core at the VA San Diego Healthcare System/Veterans Medical Research Foundation (VASDHS/VMRF) using a FACSCanto Flow Cytometer (BD Biosciences, San Jose, CA) or an iCys Research Imaging Cytometer (CompuCyte corporation, Westwood, MA). The cell cycle analysis was performed using the BD DIVA Software and the ModFit LT Software from Verity Software House, Inc. The data were analysed using the iCyte Cytometric Analysis Software with an iNovator Toolkit. Blood chemistry analysis Basic metabolic and lipid parameters were determined by the UCSD Murine Haematology and Coagulation Core Laboratory using serum from SRSF3HKO and WT mice. Fasting blood glucose concentrations were measured using ACCU-Check glucometer (Roche) and serum insulin using Mouse Insulin Ultrasensitive ELISA kit (ALPCO Immunoassays). Serum GH and IGF1 levels in the fed state were measured using commercial kits (Rat/Mouse growth hormone Elisa kit, Millipore and Quantikine Mouse/Rat IGF-1 imunoassay, R&D Systems). Measurement of liver glycogen, cholesterol and TGs Liver glycogen was measured using Glycogen Assay Kit (BioVision Research Products, Mountain View, CA) according to the manufacturer’s instructions. Livers from SRSF3HKO and WT mice were minced in PBS containing 1% triton-X. Hepatic cholesterol and TGs were measured using commercial kits (Cholesterol E and Triglyceride ELISA Kit, LabAssay from Wako Chemicals USA) following the manufacturer’s instructions. Fatty acid oxidation in liver homogenates The released 14 CO 2 and radiolabelled acid-soluble materials produced from oxidation of [1- 14 C]palmitate were measured by adapting a method published by Bandyopadhyay et al. [52] In brief, 40 μl of the homogenate (100 μg protein) or mitochondrial suspension (50 μg protein) was preincubated at 30 °C for 15 min inside a vial with a conical insert. A 160-μl reaction mixture was then added to the preincubated suspension, followed by 0.1 μCi [1- 14 C]palmitate (0.5 μCi ml −1 , final concentration 200 μmol l −1 ) as albumin complex (fatty acid and albumin dilution of 5:1). After 60 min of incubation, the reactions were stopped with HClO 4 , released radiolabelled CO 2 was trapped in an organic solvent mixture, and the radioactivity in the trapped CO 2 and acid-soluble materials in the acidified supernatant was counted. These two radioactivities were combined, and the amount of oxidized palmitate (in nmol) was calculated from the specific activity corrected for endogenous long-chain fatty acyl-coA. Dilution of the specific activity of exogenous radiolabelled palmitate in the incubations attributable to the increase in long-chain fatty acyl content in type 2 samples was minimized to 6–8% by the addition of a 10-fold excess of palmitate. The results are presented as nanomoles of palmitate oxidized per microgram protein. Glucose tolerance and insulin tolerance test To assess glucose tolerance, we fasted 3-month-old WT and HKO mice for 6 h. Blood glucose concentrations were measured by tail bleeding using an ACCU-Check glucometer, at time 0 and indicated times thereafter, for a total of 2 h, after an intraperitoneal (i.p.) injection of glucose of 1 g kg −1 body weight. For ITTs, 3-month-old mice were fasted for 4 h and insulin used for i.p. injection was 0.5 U kg −1 body weight. Mouse exon arrays Total RNA from liver tissues of the three SRSF3HKO and age-matched WT mice was isolated using an RNeasy Kit (QIAGEN). RNA quality was assessed by using the Agilent Model 2100 Bioanalyzer (Agilent Technologies). Microarray analysis was performed using GeneChip Mouse Exon 1.0 ST Arrays (Affymetrix, Santa Clara, CA). Details of analyses are described in Supplementary Methods . Microarray data are available at GEO Accession Number GSE35686 . Confirmation of altered exon utilization and gene expression Total RNA was reverse transcribed using random hexamers with MultiScribe MuLV reverse transcriptase (Applied Biosystems) then subjected to PCR using GoTaq polymerase (Promega). For confirmation of exon skipping, RT–PCR was done on each sample using primers on constitutive exons flanking the altered exon. To ensure a linear PCR amplification allowing semiquantitative assessment of the spliced products, we performed PCR analysis with 25 cycles. Representative results for two mice from each group (WT and SRSF3 HKO) are shown in the figures. PCR products were separated on 3% agarose or 12% non-denaturing polyacrylamide gels, stained with ethidium bromide, visualized and quantified with Kodak Electrophoresis Documentation and Analysis System (EDAS) 290. For the analysis of Xbp1 mRNA splicing, RT–PCR was performed with GoTaq polymerase as before, then the PCR reaction products were digested by Pst I to cut the unspliced fragment and separated by 2% agarose gel electrophoresis. For mRNA expression studies, real-time qRT–PCR assays were performed for each sample in triplicate in a final reaction volume of 20 μl. The endogenous housekeeping gene Gapdh or the gene of interest was amplified using 20 ng of cDNA with iTaq SYBR Green supermix with ROX (Bio-Rad Laboratories) on Chromo4 Thermal Cyclers (Bio-Rad). The data were analysed using the ΔΔCt method and presented as the relative change in gene expression, normalized to Gapdh . All primers for qPCR were designed with Universal Probe Library (Roche) and listed in Supplementary Table S10 . Construction and assays of splicing reporter For testing the effect of SRSF3 on Ern1 exon 13 splicing, the genomic region of mouse Ern1 exon 13 flanking 300 nt intronic regions was amplified from control liver DNA by PCR with primers listed in Supplementary Table S9 using Pfu Turbo DNA Polymerase (Stratagene). The PCR product was subcloned into a splicing reporter construct derived from human insulin receptor, minigene S [32] in place of exon 11 and surrounding introns and confirmed by sequencing. The expression vector and minigene IE was transfected into NIH3T3 cell lines. The corresponding empty vector was used as a control. Total RNA was collected 48 h after transfection using RNAzol B (Tel-Test Inc, Friendswood, TX). Total RNA (1 μg) was reverse transcribed using oligo-dT (Applied Biosystem, Foster City, CA). The transfected minigene transcripts were amplified using plasmid-specific primer pairs as described previously [32] . Histochemistry, immunohistochemistry and immunoblotting Collected tissues were fixed in 10% neutral-buffered formalin for 12 h before embedding in paraffin and staining with haematoxylin and eosin using standard procedures. In case of CD45 and Oil-Red-O staining, liver tissues were frozen directly in OCT compound. For glycogen accumulation, liver sections were stained using the periodic acid-Schiff reaction. TUNEL staining was carried out using ApopTag Peroxidase In Situ Apoptosis Detection Kit (Millipore). All histology and immunohistochemistry were performed by the UCSD Histology and Immunohistochemistry Shared Resource. For immunoblotting, livers or primary hepatocytes were lysed in extraction buffer (20 mM Tris, pH 7.9; 300 mM NaCl; 1% Nonidet P-40) supplemented with protease and phosphatase inhibitors. Liver/hepatocyte lysates were separated by SDS–PAGE, transferred to PVDF membranes and immunoblotted with primary antibodies followed by HRP-conjugated secondary antibodies and developed using an ECL+ kit (GE). List of antibodies are provided in Supplementary Methods . Dual energy X-ray absorptiometry scan Following anaesthesia with isoflurane, overnight fasted mice underwent dual energy X-ray absorptiometry scanning to measure total tissue and fat mass and lean body mass using a PixiMus mouse densitometer (GE Healthcare). Statistical analysis Data are presented as mean±s.e.m. Data were subjected to statistical analysis by ANOVA or Student’s two-tailed t -test for individual comparisons. Frequency of genotypes was analysed using Fisher’s exact test or χ 2 -test. A statistically significant difference was defined as * P <0.05, ** P <0.01, *** P <0.001, **** P <0.0001. Accession codes: Microarray data have been deposited in Gene Expression Omnibus under accession code GSE35686 . How to cite this article: Sen, S. et al. Splicing factor SRSF3 is crucial for hepatocyte differentiation and metabolic function. Nat. Commun. 4:1336 doi: 10.1038/ncomms2342 (2013).